Gut microbiome development along the colorectal adenoma–carcinoma sequence Colorectal cancer, a commonly diagnosed cancer in the elderly, often develops slowly from benign polyps called adenoma. The gut microbiota is believed to be directly involved in colorectal carcinogenesis. The identity and functional capacity of the adenoma- or carcinoma-related gut microbe(s), however, have not been surveyed in a comprehensive manner. Here we perform a metagenome-wide association study (MGWAS) on stools from advanced adenoma and carcinoma patients and from healthy subjects, revealing microbial genes, strains and functions enriched in each group. An analysis of potential risk factors indicates that high intake of red meat relative to fruits and vegetables appears to associate with outgrowth of bacteria that might contribute to a more hostile gut environment. These findings suggest that faecal microbiome-based strategies may be useful for early diagnosis and treatment of colorectal adenoma or carcinoma. Colorectal cancer (CRC) is among the top three most frequently diagnosed cancer worldwide and a leading cause of cancer mortality [1] , [2] . The incidence is higher in more developed countries, but is rapidly increasing in historically low risk areas such as Eastern Asia, Spain and Eastern Europe, attributable to a so-called western lifestyle [1] , [2] , [3] . Genetic changes accumulate for many years in the development of colorectal cancer, often involving loss of the tumour suppressor gene adenomatous polyposis coli ( APC ), followed by activating and inactivating mutations in KRAS , PIK3CA and TP53 (refs 3 , 4 ). Most CRC cases are sporadic, but are preceded by dysplastic adenomas which could progress into malignant forms, referred to as the adenoma–carcinoma sequence [3] . CRC is among the most studied diseases implicated with the gut microbiota. Causal relationships, however, were typically investigated by application of antibiotic cocktails that eradicate the gut microbiota without knowing the exact microbial strains and genes at play [5] , [6] , [7] . Fusobacterium has been detected in colorectal carcinoma relative to normal colon tissue [8] , [9] , and was found to be enriched in adenomas [10] . Fusobacterium nucleatum , a periodontal pathogen, has been shown to promote myeloid infiltration of intestinal tumours in Apc Min/+ mice and associate with increased expression of proinflammatory genes such as Ptgs2 ( COX-2 ), Scyb1 ( IL8 ), Il6 , Tnf ( TNFα ) and Mmp3 in mice and humans [11] . It is not clear, however, whether more bacteria or archaea serve as markers for, or contribute to the aetiology of, colorectal carcinomas. Moreover, as perhaps the most important environmental factor for human health, or our ‘other genome’ [12] , [13] , it remains to be explored whether and how the gut microbiome integrate other risk factors, for example, diet, smoking, obesity [1] , [2] , [3] , [14] , [15] and generate a coherent signal for colorectal carcinogenesis. Here, we present 156 metagenomic shotgun-sequenced faecal samples from colorectal adenoma and carcinoma patients and healthy controls, identify metagenomic linkage groups (MLG) [16] characteristic of the tumours, and reveal the possible impact of various risk factors, especially red meat versus fruit and vegetable consumption on gut microbial alterations along the colorectal adenoma–carcinoma sequence. Global shifts in the gut microbiome To investigate changes in the gut microbiome in colorectal adenoma and carcinoma, we performed metagenomic shotgun sequencing on 156 faecal samples from healthy controls, advanced adenoma, or carcinoma patients ( Supplementary Data 1 ). The high-quality sequencing reads (5 GB per sample on average, Supplementary Data 2 ) were assembled de novo , and the genes identified were compiled into a non-redundant catalogue of 3.5 million genes, which allowed on average 76.3% of the reads in each sample to be mapped. We first investigated the richness and evenness of the gut microbiota in the three groups ( Fig. 1 ). Rarefaction analysis based on the starting cohort of 55 healthy controls, 42 advanced adenoma and 41 carcinoma patients showed that the gene richness approached saturation in each group, and is higher in advanced adenoma than in control, and higher in carcinoma than in advanced adenoma ( Fig. 1a ). Both gene and genus richness were significantly different among the three groups ( P =0.005, P =3.2e–7, respectively, Kruskal–Wallis test; Fig. 1b,e ), while the α-diversities were not ( Fig. 1c,f ), consistent with previous 16S ribosomal RNA gene pyrosequencing analysis on adenoma and healthy controls [17] . The number of virulence genes according to the virulence factor database [18] also significantly differed among the groups ( P =1.2e–5, Kruskal–Wallis test; Fig. 1d , Supplementary Data 3 ). Thus, greater richness in genes or genera is not a sign of a healthy gut microbiota in this cohort, but likely indicates overgrowth of a variety of harmful bacteria or archaea in patients with advanced colorectal adenoma or carcinoma. 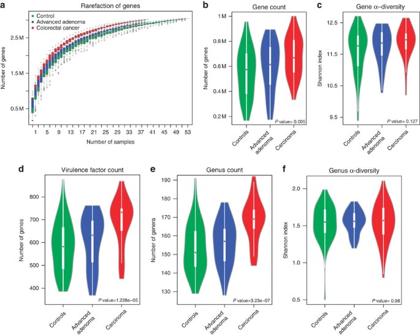Figure 1: Increased gut microbiome richness in CRC. (a) Rarefaction for gut microbial gene content in healthy, advanced adenoma and carcinoma samples56. The number of genes in each group was calculated after 100 random sampling with replacement. Plotted are interquartile ranges (IQRs; boxes), medians (dark lines in the boxes), the lowest and highest values within 1.5 times IQR from the first and third quartiles (whiskers above and below the boxes), and outliers beyond the whiskers (circles). (b,c) Richness and α-diversity (Shannon index) of the three cohorts at the gene level. Violin plots showing both the richness or diversity values and their density. (d) Richness of genes encoding virulence factors18(Supplementary Data 3). (e,f) Richness and α-diversity (Shannon index) of the three cohorts at the genus level.n=55 healthy controls, 42 advanced adenoma and 41 carcinoma patients.Pvalues from Kruskal–Wallis tests are shown. Figure 1: Increased gut microbiome richness in CRC. ( a ) Rarefaction for gut microbial gene content in healthy, advanced adenoma and carcinoma samples [56] . The number of genes in each group was calculated after 100 random sampling with replacement. Plotted are interquartile ranges (IQRs; boxes), medians (dark lines in the boxes), the lowest and highest values within 1.5 times IQR from the first and third quartiles (whiskers above and below the boxes), and outliers beyond the whiskers (circles). ( b , c ) Richness and α-diversity (Shannon index) of the three cohorts at the gene level. Violin plots showing both the richness or diversity values and their density. ( d ) Richness of genes encoding virulence factors [18] ( Supplementary Data 3 ). ( e , f ) Richness and α-diversity (Shannon index) of the three cohorts at the genus level. n =55 healthy controls, 42 advanced adenoma and 41 carcinoma patients. P values from Kruskal–Wallis tests are shown. Full size image Enterotype, another general measure of the gut microbiota [19] , [20] , divided the cohort into two or three clusters (depending on the method used, Fig. 2a,b , Supplementary Fig. 1a ), each containing healthy controls, adenoma and carcinoma patients. Yet, a greater percentage of carcinoma and adenoma patients were seen with the enterotype containing a high level of Bacteroides , while more healthy samples were found in the enterotype represented by Ruminococcus ( Fig. 2c,d , Supplementary Fig. 1b,c ). Neither the original partitioning around medoid (PAM) clustering method [19] nor the Dirichlet multinomial mixture model-based method [20] detected a Prevotella -dominated enterotype, in agreement with population-specific features or continuity of enterotypes [21] . The analyses confirmed profound shifts in the gut microbiota before or during the development of colorectal cancer. 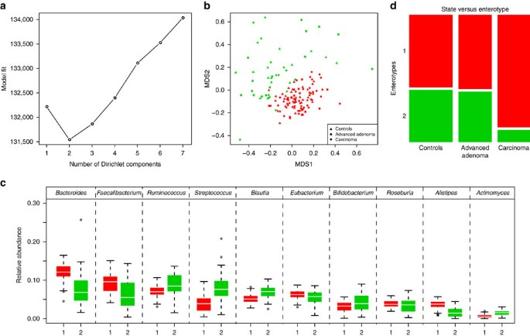Figure 2: Difference in community types. (a) Fitting to the DMM model20indicates optimal classification into two community types. (b) Plot for non-metric dimensional scaling (NMDS) ordination of Jensen–Shannon divergence values between stool samples using DMM. Red, community type 1; green, community type 2. (c) Relative abundances of the top 10 most abundant genera in the two community types. Box plot as inFig. 1a. (d) Distribution of the healthy control, advanced adenoma and carcinoma samples in the community types. The areas of the columns scale with sample size, that is,n=55, 42 and 41, respectively.P=0.00072, Fisher test;P=0.0014,χ2-test. Figure 2: Difference in community types. ( a ) Fitting to the DMM model [20] indicates optimal classification into two community types. ( b ) Plot for non-metric dimensional scaling (NMDS) ordination of Jensen–Shannon divergence values between stool samples using DMM. Red, community type 1; green, community type 2. ( c ) Relative abundances of the top 10 most abundant genera in the two community types. Box plot as in Fig. 1a . ( d ) Distribution of the healthy control, advanced adenoma and carcinoma samples in the community types. The areas of the columns scale with sample size, that is, n =55, 42 and 41, respectively. P =0.00072, Fisher test; P =0.0014, χ 2 -test. Full size image MLGs characteristic of adenoma or carcinoma To explore signatures of the gut microbiome in healthy or tumour samples, we identified 130,715 genes that displayed significant abundance differences in any two of the three groups (Kruskal–Wallis test, Benjamin–Hochberg q -value<0.1; Fig. 3 ). None of the available phenotypes other than tumour status displayed a significant difference among the controls, adenoma and carcinoma patients, except for serum ferritin and red meat consumption ( P <0.05, Kruskal–Wallis test, Supplementary Data 4 ). About 58.9% of the gene markers were significantly elevated in carcinoma compared with both healthy and advanced adenoma samples ( Fig. 3a ), indicating that they were specific to colorectal cancer; another 24.3% of the genes were significantly more abundant in carcinomas than controls, with intermediate levels in advanced adenomas. Among the genes with a descending trend, 5,388 (4.1% of total) were significantly reduced in carcinoma compared with both healthy and advanced adenoma samples; 2,601 (2.0% of total) were significantly less abundant in carcinomas than controls, with intermediate levels in advanced adenomas. These control-enriched genes were more often mapped to Kyoto Encyclopedia of Genes and Genomes (KEGG) pathways than the adenoma- or carcinoma-enriched genes ( Fig. 3b ). The disparity in the number of increasing and decreasing genes suggests that the increase in pathobionts is more pronounced than the decrease in beneficial bacteria during the development of carcinoma. 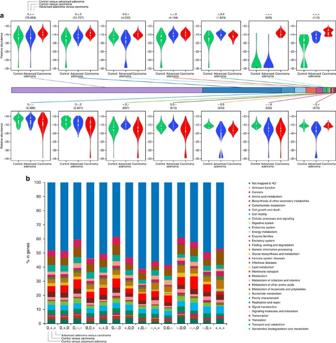Figure 3: Gene markers along the adenoma–carcinoma sequence. (a) All 130,715 differentially enriched genes (Benjamin–Hochbergq-value<0.1) were grouped according to their direction of enrichment in control versus adenoma, control versus carcinoma and adenoma versus carcinoma, where + indicates enrichment in latter, − indicates enrichment in former and 0 indicates no difference (p≥0.05, Wilcoxon rank-sum test, Bonferroni correction to control for multiple testing). The relative abundance of genes in each group is shown in violin plot, that is, interquartile ranges (IQRs; thick bars), medians (open dots on the bars), the lowest and highest values within 1.5 times IQR from the first and third quartiles (lines above and below the bars) and density of values (width between curves). The number of genes in each group is shown in parenthesis and as coloured blocks on the central bar. (b) Distribution in KEGG level 2 pathways of the gene markers ina. Figure 3: Gene markers along the adenoma–carcinoma sequence. ( a ) All 130,715 differentially enriched genes (Benjamin–Hochberg q -value<0.1) were grouped according to their direction of enrichment in control versus adenoma, control versus carcinoma and adenoma versus carcinoma, where + indicates enrichment in latter, − indicates enrichment in former and 0 indicates no difference ( p ≥0.05, Wilcoxon rank-sum test, Bonferroni correction to control for multiple testing). The relative abundance of genes in each group is shown in violin plot, that is, interquartile ranges (IQRs; thick bars), medians (open dots on the bars), the lowest and highest values within 1.5 times IQR from the first and third quartiles (lines above and below the bars) and density of values (width between curves). The number of genes in each group is shown in parenthesis and as coloured blocks on the central bar. ( b ) Distribution in KEGG level 2 pathways of the gene markers in a . Full size image The significantly different genes were clustered into MLGs according to their abundance co-variations among all samples, which allowed identification of microbial species characteristic of each group [16] . A number of Bacteroides and Parabacteroides species, along with Alistipes putredinis , Bilophila wadsworthia , Lachnospiraceae bacterium and Escherichia coli were enriched in carcinoma samples compared with both healthy and advanced adenoma samples ( Fig. 4 , Supplementary Data 5 ). The likely oral anaerobes mlg-75, mlg-83, mlg-84, mlg-88 (related to Fusobacterium sp. oral taxon 370, Pavimonas micra , Gemella morbillorum and Peptostreptococcus stomatis , respectively) and mlg-77 formed a cluster of positive correlations relatively separate from other carcinoma-enriched MLGs ( Fig. 4b,c ). mlg-75, mlg-88 and mlg-77 were also elevated in adenoma compared with control samples ( Fig. 4a ). Gut commensals such as Bifidobactium animalis and Streptococcus thermophilus , on the other hand, decreased in faeces from adenoma or carcinoma patients, consistent with deviation from a healthy microbiome. 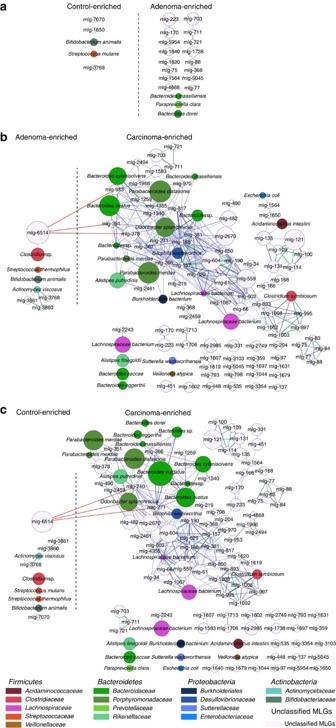Figure 4: Gut MLGs in the controls, advanced adenoma or carcinoma samples. (a) Control versus advanced adenoma (n=55 and 42). (b) Advanced adenoma versus carcinoma (n=42 and 41). (c) Control versus carcinoma (n=55 and 41). For all MLGs containing >100 genes, the direction of enrichment was determined by Wilcoxon rank-sum test (P<0.05,Supplementary Data 3). Size of the nodes scales with the number of genes (102~3613) in the MLG. MLGs annotated to species or genera are coloured according to family. Edges between nodes indicate Spearman’s correlation >0.8 (green), between 0.6 and 0.8 (light to dark blue) or <−0.6 (red), calculated according to the samples under comparison. Figure 4: Gut MLGs in the controls, advanced adenoma or carcinoma samples. ( a ) Control versus advanced adenoma ( n =55 and 42). ( b ) Advanced adenoma versus carcinoma ( n =42 and 41). ( c ) Control versus carcinoma ( n =55 and 41). For all MLGs containing >100 genes, the direction of enrichment was determined by Wilcoxon rank-sum test ( P <0.05, Supplementary Data 3 ). Size of the nodes scales with the number of genes (102~3613) in the MLG. MLGs annotated to species or genera are coloured according to family. Edges between nodes indicate Spearman’s correlation >0.8 (green), between 0.6 and 0.8 (light to dark blue) or <−0.6 (red), calculated according to the samples under comparison. Full size image In agreement with the MLGs, genera including Ruminococcus , Bifidobacterium and Streptococcus were significantly overrepresented in the controls, while Bacteroides , Alistipes , Escherichia , Parvimonas , Bilophila and Fusobacterium were overrepresented in the carcinoma patients ( Supplementary Fig. 2 ). E. coli , mlg-331, mlg-711 and mlg-1607 were more abundant in samples histologically determined as carcinoma in situ compared with samples from adenocarcinoma, whereas mlg-75, mlg-83, mlg-84 and mlg-1697 were more abundant in adenocarcinoma ( P <0.05, Wilcoxon rank-sum test, False discovery rate (FDR)=0.7216; Supplementary Fig. 3 ). Seven of the 126 MLGs (containing over 100 genes) exhibited significant differences among carcinoma stages [22] ( P <0.05, Kruskal–Wallis test, FDR=0.531), often peaking in Stage II or III ( Supplementary Fig. 4 ). Many of the carcinoma-associated MLGs were more abundant in samples from patients with carcinoma in the rectum or left colon (the splenic flexure, descending colon and sigmoid colon) than in the right colon (the caecum, ascending colon and transverse colon) ( Supplementary Fig. 5 ), indicating that faeces were best proxy for the environment at the end of the gastrointestinal tract, yet could still reveal malignancy at the beginning of the colon. MLG-based classification of adenoma or carcinoma To illustrate diagnostic value of the faecal microbiome for colorectal cancer, we constructed a random forest classifier that could detect carcinoma samples. Five repeats of 10-fold cross-validation (that is, 50 tests) in the training set consisted of 55 controls and 41 carcinoma samples led to the optimal selection of 15 MLG markers that performed nicely on the training set ( Fig. 5a–c , Supplementary Data 1 and 5 ). The classification error remained low on the test set (8 controls, 47 advanced adenomas and 5 carcinomas), showing an area under receiver operating curve (AUC) of 96% (advanced adenoma considered as non-carcinoma, Fig. 5d,e , Supplementary Data 1 ). Including age and body mass index (BMI) together with the 126 MLGs did not change the markers selected. Consistently, most of the MLGs were similarly enriched in (AUC) elderly and middle-aged subjects (above and below 65 years old; Supplementary Fig. 6 , Supplementary Data 5 ), indicating common characteristics of the carcinoma-associated gut microbiome. 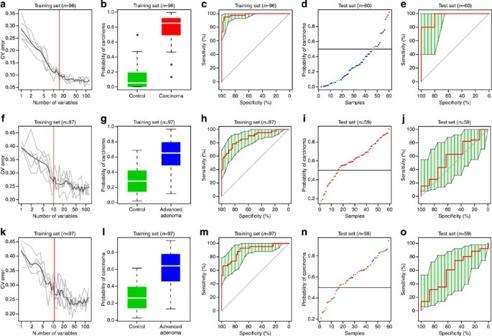Figure 5: Gut MLGs classify colorectal carcinoma and adenoma samples from healthy controls. (a) Distribution of 5 trials of 10-fold cross-validation error in random forest classification of carcinoma as the number of MLGs increases. The model was trained using relative abundance of the MLGs (>100 genes) in the controls and carcinoma samples (n=55 and 41). The black curve indicates average of the five trials (grey lines). The pink line marks the number of MLGs in the optimal set (Supplementary Data 5). The same MLGs were selected if age and BMI were included along with the MLGs. (b) Box-and-whisker plot for the probability of carcinoma in the cross-validational training set according to the model ina. (c) Receiver operating curve (ROC) for the training set. The area under receiver operating curve (AUC) is 98.34% and 95% confidence interval (CI) is 96.29–100%. (d) Classification of the test set consisted of 8 controls (green), 47 advanced adenoma (blue) and 5 carcinoma (red), that is, 18 unused samples and 42 adenoma samples used in analyses inFigs 1,2,3,4,6and7. (e) ROC for the test set. The AUC is 96% and 95% CI is 87.88–100%. (f–j) Training and testing the model that classifies adenomas from controls, performed as ina–e. The AUC for the training set (n=55 controls, 42 adenomas) is 87.38% and 95% CI is 80.21–94.55%; the AUC for the test set (8 controls, 5 advanced adenomas and 46 carcinomas) is 59.56% and 95% CI is 37.51–81.61%. (k–o) Training and testing the model that classifies adenomas from controls, performed as in (f–j) except that age and BMI were included along with the MLGs. Age was selected by the model, making the optimal number of markers 11. The AUC for the training set is 89.74% and 95% CI is 83.32–96.16%; the AUC for the test set is 59.56% and 95% CI is 37.64–81.48%. Figure 5: Gut MLGs classify colorectal carcinoma and adenoma samples from healthy controls. ( a ) Distribution of 5 trials of 10-fold cross-validation error in random forest classification of carcinoma as the number of MLGs increases. The model was trained using relative abundance of the MLGs (>100 genes) in the controls and carcinoma samples ( n =55 and 41). The black curve indicates average of the five trials (grey lines). The pink line marks the number of MLGs in the optimal set ( Supplementary Data 5 ). The same MLGs were selected if age and BMI were included along with the MLGs. ( b ) Box-and-whisker plot for the probability of carcinoma in the cross-validational training set according to the model in a . ( c ) Receiver operating curve (ROC) for the training set. The area under receiver operating curve (AUC) is 98.34% and 95% confidence interval (CI) is 96.29–100%. ( d ) Classification of the test set consisted of 8 controls (green), 47 advanced adenoma (blue) and 5 carcinoma (red), that is, 18 unused samples and 42 adenoma samples used in analyses in Figs 1 , 2 , 3 , 4 , 6 and 7 . ( e ) ROC for the test set. The AUC is 96% and 95% CI is 87.88–100%. ( f – j ) Training and testing the model that classifies adenomas from controls, performed as in a – e . The AUC for the training set ( n =55 controls, 42 adenomas) is 87.38% and 95% CI is 80.21–94.55%; the AUC for the test set (8 controls, 5 advanced adenomas and 46 carcinomas) is 59.56% and 95% CI is 37.51–81.61%. ( k – o ) Training and testing the model that classifies adenomas from controls, performed as in ( f – j ) except that age and BMI were included along with the MLGs. Age was selected by the model, making the optimal number of markers 11. The AUC for the training set is 89.74% and 95% CI is 83.32–96.16%; the AUC for the test set is 59.56% and 95% CI is 37.64–81.48%. Full size image Among the MLG markers were the likely oral anaerobes mlg-75 and mlg-84, the former also showed a high odds ratio for adenoma ( Supplementary Data 5 ), suggesting an early role in pathogenesis. Other MLG markers included Bacteroides massiliensis , mlg-2985, mlg-121 and ten more taxonomically undefined MLGs ( Supplementary Data 5 ). Thus, MLGs selected by the carcinoma classifier captured important features of the deteriorating gut microbiome in adenoma and carcinoma and have great potential for early and non-invasive diagnosis of these tumours. We directly investigated the utility of the gut MLGs for identifying adenoma, which is more difficult to screen than colorectal carcinoma but important for early intervention [3] , [23] . After five repeats of 10-fold cross-validation, the random forest model chose 10 MLGs that allowed optimal classification of the training set (55 controls and 42 advanced adenoma; Fig. 5f–h , Supplementary Data 1 and 5 ). On the test set (8 controls, 5 advanced adenoma and 46 carcinoma), all the advanced adenoma samples were correctly classified, while performance on the control and carcinoma samples were not as satisfactory (carcinoma considered as adenoma positive, Fig. 5i,j , Supplementary Data 1 ). When age and BMI were included along with the 126 MLGs, age was selected as a marker together with the 10 MLGs ( Fig. 5k–m ), but performance on the test set did not improve ( Fig. 5n,o ). Therefore, the faecal MLGs offer new opportunities for non-invasive detection of colorectal adenoma as well as carcinoma, but additional examinations would probably be necessary for confirming adenoma. Diet-associated functional changes in the microbiome Dietary components such as red meat are known risk factors for colorectal carcinoma [3] , [14] , [15] , but it is not known how diet makes a footprint on gut microbes associated with or even causing colorectal carcinoma. We assessed influence of a number of clinical or lifestyle factors on gut microbial genes or MLGs, and found that the control, adenoma or carcinoma state was indeed among the strongest factors ( Supplementary Fig. 7a , Supplementary Data 6 ). Interestingly, the influence of fruit and vegetable consumption pointed towards control-enriched MLGs in canonical coordinate analysis (CCA), while C-reactive protein (CRP) and meat consumption were associated with carcinoma-enriched MLGs ( Supplementary Fig. 7a ). Spearman’s correlation coefficient of ≥0.2 was observed between relative abundance of the MLGs and the dietary or physiological parameters ( Fig. 6 , Supplementary Figs 8 and 9 ). Carcinoma-enriched bacteria that produce short chain fatty acids, the major energy source for colonocytes, through amino acid fermentation, and/or bacteria that metabolize bile acids [24] , [25] , for example, B. massiliensis , B. dorei , B. vulgates , Parabacteroides merdae , A. finegoldii and B. wadsworthia , showed a positive correlation with consumption of red meat and/or a negative correlation with consumption of fruits and vegetables ( Fig. 6 ), suggesting a common pathway in colorectal tumourigenesis. The control-enriched MLGs S. mutans and Clostridium sp., on the other hand, positively correlated with vegetable intake. These weak correlations with diet were supported by significant differences in the MLGs between high and low intake groups ( Supplementary Fig. 7b–h ). Carcinoma-enriched bacteria such as B. massiliensis , P. merdae , A. finegoldii and B. wadsworthia were less abundant in subjects consuming more vegetable or fruits, in contrast to the control-enriched S. mutans and Clostridium sp. ( Supplementary Fig. 7b,d ). Carcinoma MLGs including mlg-84, mlg-850 and mlg-1738 were more abundant in subjects consuming a greater amount of total meat or red meat ( Supplementary Fig. 7e,f ). 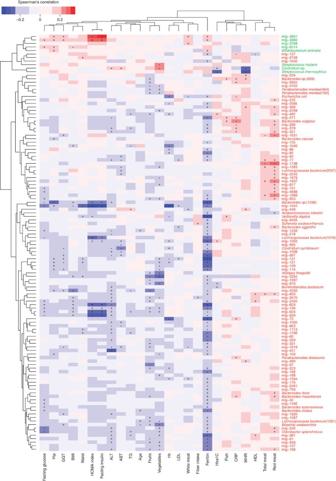Figure 6: Numerical correlation between dietary or clinical indices and MLGs. Spearman’s correlation coefficient was calculated between the relative abundance of each MLG (>100 genes) and the level of risk factors or clinical phenotypes indicated. Red, positive correlation; blue, negative correlation. +,P<0.05, FDR=0.4131; *,P<0.01, FDR=0.2635. The name of each MLG was coloured according to its direction of enrichment, that is, green if higher in controls than in carcinomas, red if higher in carcinomas than in controls.Actinomyces viscosus,Alistipes putredinis,Paraprevotella clara, mlg-703, mlg-711, mlg-798, mlg-1602 and mlg-7070 did not have significant correlations with any of the 26 numerical phenotypes (P>0.05, Spearman’s) and are not shown. gamma-glutamyl transferase (GGT), body mass index (BMI), alanine transaminase (ALT), aspartate transaminase (AST), triglyceride (TG), haemoglobin (Hb), low density lipoprotein (LDL), C-reactive protein (CRP), waist–hip ratio (WHR), high density lipoprotein (HDL). Figure 6: Numerical correlation between dietary or clinical indices and MLGs. Spearman’s correlation coefficient was calculated between the relative abundance of each MLG (>100 genes) and the level of risk factors or clinical phenotypes indicated. Red, positive correlation; blue, negative correlation. +, P <0.05, FDR=0.4131; *, P <0.01, FDR=0.2635. The name of each MLG was coloured according to its direction of enrichment, that is, green if higher in controls than in carcinomas, red if higher in carcinomas than in controls. Actinomyces viscosus , Alistipes putredinis , Paraprevotella clara , mlg-703, mlg-711, mlg-798, mlg-1602 and mlg-7070 did not have significant correlations with any of the 26 numerical phenotypes ( P >0.05, Spearman’s) and are not shown. gamma-glutamyl transferase (GGT), body mass index (BMI), alanine transaminase (ALT), aspartate transaminase (AST), triglyceride (TG), haemoglobin (Hb), low density lipoprotein (LDL), C-reactive protein (CRP), waist–hip ratio (WHR), high density lipoprotein (HDL). Full size image Serum levels of ferritin, a protein responsible for intracellular iron storage, negatively correlated with many of the carcinoma-enriched MLGs ( Fig. 6 ), highlighting iron as a key resource for the growth of a number of pathogenic bacteria [26] , which feed on iron from the host or dietary sources such as meat. Haemoglobin (Hb) displayed negative correlation with the carcinoma-enriched mlg-75, mlg-2985, mlg-88 and mlg-84. Other known risk factors, such as current or ever smoking also coincided with enrichment of MLGs (including B. dorei and B. vulgatus ; Supplementary Figs 8 and 9 ). Waist–hip ratio negatively correlated with the control-enriched Clostridium sp. and S. thermophilus , and positively correlated with the carcinoma-enriched Bacteroides sp., mlg-368 and mlg-448 ( Fig. 6 ). BMI, on the other hand, showed negative correlation with some carcinoma-enriched MLGs. These results are in agreement with meta-analysis showing that central obesity is a more reliable risk factor for CRC than general obesity [27] . Consistent with a significant role played by diet, KEGG orthology (KO) modules for phosphotransferase systems, transporters for a number of different sugars, were overrepresented in healthy controls compared with adenoma samples or in adenoma compared with carcinoma samples ( Fig. 7 , Supplementary Data 7 ). Modules for transporting the amino acids histidine, arginine and lysine were enriched in carcinoma compared with adenoma, whereas those for synthesizing histidine, lysine, methionine, cysteine, leucine and tryptophan were enriched in control compared with adenoma, or adenoma compared with carcinoma samples. Besides increased capacity for the utilization of dietary or host amino acids along the adenoma–carcinoma sequence, increased capacity for metabolizing host glycans such as mucin and glycosaminoglycans was suggested by the higher abundance of KO modules for the degradation of dermatan sulphate, heparin sulphate and keratan sulphate ( Fig. 7 ). The sulfatases in these modules have been characterized in Flavobacterium heparinum , B. thetaiotaomicron and seen in other Bacteroides [28] , [29] , [30] , [31] . Sulfonate/nitrate/taurine transport system was elevated in adenomas compared with controls, suggesting changes in the metabolism of bile acids ( Fig. 7 , Supplementary Data 7 ). Higher levels of methanogenesis modules were also observed in adenomas or carcinomas compared with healthy controls. Moreover, these differentially enriched functions such as lipopolysaccharide (LPS) biosynthesis, keratan sulphate degradation and iron(III) transport system could be found in the MLG markers in the classifier for adenoma or carcinoma, along with more house-keeping functions ( Fig. 7 , Supplementary Data 8–10 ). Together, our results suggest venues through which a diet low in fruits and vegetables relative to meats select for outgrowth of putrefactive bacteria, which might help promote colorectal carcinoma. 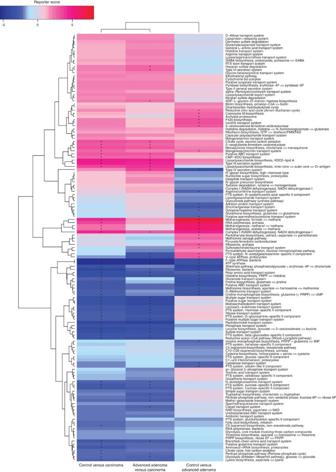Figure 7: KO modules overrepresented in healthy controls, colorectal adenoma or carcinoma samples. The relative abundances of KO modules were compared between control and adenoma, adenoma and carcinoma, or control and carcinoma, and modules with a significant difference in reporter score (<−1.7, enriched in former; >1.7, enriched in latter) are shown. +, reporter score >2.3 or <−2.3. Figure 7: KO modules overrepresented in healthy controls, colorectal adenoma or carcinoma samples. The relative abundances of KO modules were compared between control and adenoma, adenoma and carcinoma, or control and carcinoma, and modules with a significant difference in reporter score (<−1.7, enriched in former; >1.7, enriched in latter) are shown. +, reporter score >2.3 or <−2.3. Full size image In addition to functions listed in the KEGG database, the gut microbiota have been reported to control response to cancer therapies [6] , [32] . Alistipes and Ruminococcus positively correlated with TNF production after anti-IL-10R/CpG oligonucleotide immunotherapy in C57Bl/6 mice transplanted with MC38 colon carcinoma [6] . We observed increase in A. finegoldii , mlg-482 (most related to A. onderdonkii ), A. putredinis in colorectal carcinoma and decrease in mlg-6514 (most related to Ruminococcus sp. 5_1_39BFAA) whose abundance anti-correlated with a few carcinoma-enriched MLGs ( Fig. 4b,c , Supplementary Data 5 ). All these MLGs were present in close to 100% of the carcinoma patients regardless of histology, stage or location of the tumour. P. distasonis monoassociation had been shown to compromise immunogenic chemotherapy by doxorubicin against established MCA205 sarcomas in mice [32] . MLGs for P. distasonis and P. merdae were more abundant in carcinoma than advanced adenoma samples, and were detected in most carcinoma samples ( Fig. 4b,c , Supplementary Data 5 ). Collectively, these results indicate that gut microbes present or overgrown in human colorectal carcinoma might facilitate or abrogate immuno or chemotherapies, and should be examined for optimal selection of treatment plans for each patient. In summary, our metagenome-wide association study for the gut microbiome of healthy controls, colorectal adenoma and carcinoma patients identified genes, strains (MLGs) and functions associated with the tumours, and open new ways for early detection and patient stratification of colorectal adenoma and carcinoma. It remains to be seen how our markers might help improve non-invasive screening of the colorectal tumours in larger cohorts around the world. In colitis-associated CRC mouse models, enterotoxigenic B. fragilis induces colitis and colonic tumours through a T helper type 17 (Th17) inflammatory response, and adherent-invasive E. coli also promotes cancer [33] , [34] , [35] . B. ovatus and B. vulgatus have been reported to be higher in human cases of Crohn’s disease (six discordant and four concordant twin pairs) [36] . We observed significant increase of B. dorei and B. massiliensis from healthy to advanced adenoma, and significant increase of B. massiliensis , B. ovatus , B. vulgatus and E. coli from advanced adenoma to carcinoma ( Fig. 4 ). B. dorei , B. vulgatus and E. coli also correlated with levels of CRP, a marker for acute inflammation ( Fig. 6 ). These results suggest analogous roles played by gut microbes in colitis-associated and adenoma-linked CRC. Akkermansia , a mucin-degrading bacterium in the phylum of Verrucomicrobia , has been reported to correlate with CRC in humans and in a mouse model [37] , [38] . We observed no difference in the abundance of Akkermansia among healthy controls, advanced adenoma and carcinoma samples ( Supplementary Fig. 2 ). Two of the three PAM-based enterotypes contained a relatively high level of Akkermansia , which included more controls and carcinoma samples, respectively ( Supplementary Fig. 1 ). Future analyses taking into account factors such as obesity, diet and meal time would help resolve the possible role of this important bacterium in CRC. Even though putrefactive bacteria such as Alistipes and Bacteroides could produce short chain fatty acid from amino acids, carbohydrate fermentation is still preferred [24] , [39] , which might explain protective roles of fruits and vegetables. In some Fusobacterium species, however, transport of sugar depends on amino acid fermentation (Glu, Lys, His or Ser) [40] , [41] , suggesting that they only thrive in the presence of an ample supply of amino acids. Phenolic compounds are produced from fermentation of the aromatic amino acids phenylalanine and tyrosine [39] , which might increase DNA damage in the colon. Bile acid metabolism by Bacteroides species and B. wadsworthia would also affect gut microbial composition and impact host physiology [42] , [43] . B. wadsworthia , in particular, utilizes taurine-conjugated bile acids in sulphite reduction, and promotes colitis in genetically susceptible mice (Il10 −/− ) [44] . Bile acids have also been shown to cause DNA damage and promote hepatocellular carcinoma in mice [45] , [46] . Future research would help elucidate how the known risk factors like diet, obesity and smoking collectively act on the gut microbiome in the development of colorectal carcinoma. Among the control-enriched MLGs were the lactic acid-producing bacteria Bifidobacterium animalis , S. mutans and S. thermophilus . The lactic acid produced might help lower the pH and inhibit amino acid degradation in the colon [24] , [39] . Lactobacillus and Bifidobacterium have been found to stimulate NADPH oxidase 1-dependent ROS generation and intestinal stem cell proliferation [47] , and lactate was reported to accelerate colon epithelial cell turnover in starvation-refed mice [48] . Thus, advanced colorectal adenoma or carcinoma patients appear to be deficient in lactic acid-producing commensals such as Bifidobacterium that could promote daily renewal of the colon epithelium and inhibit potential pathogens. Gut microbiota-dependent dietary or lifestyle intervention against colorectal carcinoma warrants further investigation. Study cohort and patient information The study was conducted both in participants of a health screening programme according to national screening recommendations for CRC [49] as well as in patients with suspected CRC undergoing colonoscopy as part of the clinical workup at the Department of Internal Medicine, Oberndorf Hospital (Teaching Hospital of the Paracelsus Medical University Salzburg, Austria) between 2010 and 2012. The study was approved by the local ethics committee (Ethikkommission des Landes Salzburg, approval no. 415-E/1262/2-2010) and informed consent was obtained from all participants. Data from 147 Caucasians aged between 45–86 years were included in the initial analysis, including 57 healthy controls (24 females and 33 males), 44 advanced adenoma (22 females and 22 males) and 46 carcinoma (18 females and 28 males) ( Supplementary Data 1 ). Nine additional samples taken for another manuscript (six healthy controls and three advanced adenoma samples, Supplementary Data 1 ) were also used in the test sets for the MLG-based adenoma or carcinoma classifier ( Fig. 5 ). So far, no study has investigated the given topic in a comparable manner; therefore no formal power analysis for sample size calculation could be performed. However, judging from previous 16S- and metagenomic shotgun-sequencing studies on the faecal microbiota in diseases, this is a reasonable sample size. Subjects were stratified with respect to gender, age and BMI so that the three groups (control, advanced adenoma and carcinoma) were comparable with respect to these variables. In the advanced adenoma group, 14 were located to the right colon (including caecum, ascending colon and transverse colon), 15 were located to the left colon (ranging from the splenic flexure to the sigmoid) and 15 to the rectum. In the carcinoma group, 8 were located to the right colon, 11 to the left colon and 27 to the rectum. Colorectal carcinoma was classified by the American Joint Committee on Cancer (AJCC) TNM staging system [22] . Metabolic syndrome was evaluated as defined by the National Cholesterol Education Program Adult Treatment Panel [50] . Blood pressure was measured twice by a nurse after a 5-min rest in a sitting position and the average was taken as the measurement of blood pressure. Waist circumference was taken at the highest point of the iliac crest with subjects standing in an upright position. The metabolic syndrome was diagnosed when three of the following criteria were met: fasting blood glucose level ≥6.1 mmol l −1 , waist circumference >102 cm or >88 cm in males or females, respectively, blood pressure ≥130/85 mm Hg or current antihypertensive treatment, plasma triglycerides ≥1.7 mmol l −1 , plasma HDL <1.0 mmol l −1 or <1.3 mmol l −1 in males or females, respectively, or current statin therapy. BMI was calculated as weight/squared body height (kg m −2 ). Serum ferritin was measured by Architect CI 4100 Analyzer, using the ferritin chemoluminiscent microparticle assay (ABBOTT Laboratories, Abbott Europe, Delkenheim, Germany). Laboratory assessment Following an overnight fast, a venous blood sample was obtained in all subjects and analyzed by standard laboratory methods. Blood was centrifuged and plasma was analyzed for triglycerides, cholesterol, high density and low density lipoprotein cholesterol and CRP. A standardized oral glucose tolerance test was performed with 75 g of glucose in 300 ml of water. HbA1c was measured by HPLC using Adamts H-8160 (Menarini, Florence, Italy). The homoeostasis model assessment (HOMA-IR; fasting insulin (μU l −1 ) × fasting glucose (mmol dl −1 )/22.5) was used to assess insulin resistance. Type 2 diabetes was classified as use of diabetes medication or Hba1C ≥6.5% or oral glucose tolerance test >11.1 mmol l −1 after 2 h or fasting glucose >7.0 mmol l −1 . Stool samples Fresh stool samples were collected from all patients and subjects. Samples were mechanically homogenized with a sterile spatula, then four aliquots were taken, using the Sarstedt stool sampling system (Sarstedt, Nümbrecht, Germany). Each aliquot contained 1 g of stool in a sterile 12 ml cryovial. Faecal aliquots were then stored at home freezers at −20 °C and transported to the laboratory within 48 h after collection in a freezer pack, where they were immediately stored at −80 °C. Patients and subjects did not receive probiotics or antibiotics within the last 3 months. Colonoscopy The laxative Klean–Prep (containing macrogol 59.0 g, sodium sulphate 5.68 g, sodium bicarbonate 1.68 g, NaCl 1.46 g and potassium chloride 0.74 g; Norgine, Marburg, Germany) was used for bowel preparation before colonoscopy. Colonoscopic findings were classified as tubular adenoma, advanced adenoma, that is, villous or tubulovillous features, size ≥1 cm, or high-grade dysplasia or carcinoma after a combined analysis of macroscopic and histological results [51] , [52] . Lesions were classified by location (that is, right colon including caecum, ascending colon and transverse colon, left colon ranging from the splenic flexure to the sigmoid and rectum alone). Assessment of lifestyle and dietary habits A detailed medical history, including lifestyle and dietary questionnaires, was obtained. Smoking status was classified into never smokers, former smokers and current smokers (including detailed assessment of current and former smoked cigarettes per day; data reported in packs per year). Physical activity was assessed using the international physical activities questionnaire (IPAQ) [53] and subjects were grouped into three groups: low, moderate and high physical activity according to published scoring protocol. Dietary habits were assessed using a detailed standardized questionnaire within 1 week of the faecal donation and the colonoscopy. The amount of one serving as well as the fibre content was calculated according to the recommendations of the American Heart Association ( www.heart.org ). Meat consumption was asked in detail for pork, beef, veal and venison (grouped as red meat); chicken and turkey (white meat) and offal. Furthermore, the frequency and amount of the consumption of vegetables, fruits and fish were assessed and total intake of fibre was calculated. The study was approved by the local ethics committee (Ethikkommission des Landes Salzburg, approval no. 415-E/1262/2-2010) and informed consent was obtained from all participants. Metagenomic sequencing and gene catalogue construction Paired-end metagenomic sequencing was performed on the Illumina platform (insert size 350 bp, read length 100 bp), and the sequencing reads were quality controlled and de novo assembled into contigs using SOAPdenovo v2.04 (refs 16 , 54 ; default parameters except for -K 51 –M 3 -F –u). Gene prediction from the assembled contigs was performed using GeneMark v2.7d. Redundant genes were removed using BLAT [55] with the cutoff of 90% overlap and 95% identity (no gaps allowed). Relative abundances of the genes were determined by aligning high-quality sequencing reads to the gene catalogue using the same procedure as in ref. 16 . Taxonomic assignment of the predicted genes was performed according to the IMG database (v400) using an in-house pipeline [16] , with 80% overlap and 65% identity top 10% scores (BLASTN v2.2.24, -e 0.01 -b 100 -K 1 -F T -m 8). The cutoffs were 65% identity for assignment to phylum, 85% identity to genus, 95% identity to species and ≥50% consensus for the taxon under question, if multiple hits remained. Rarefaction curve Rarefaction analysis was performed to assess the gene richness in the healthy controls, advanced adenoma and carcinoma samples. For a given number of samples, we performed random sampling 100 times in the cohort with replacement and estimated the total number of genes that could be identified from these samples by the Chao2 richness estimator [56] . To minimize erroneous identification, only the genes with ≥1 pair of mapped reads were determined to be present in a sample. Quantification of virulence factors Putative amino acid sequences were aligned against the proteins in the Virulence Factors of pathogenic bacteria Databases (VFDB) [18] using BLASTP (v2.2.24, default parameter except that -p blastp -a 2 -F F -e 1e-3 -m 8). A protein was assigned to a virulence factor by the highest scoring annotated hit containing an identity >35% and high-scoring segment pair scoring >60 bits. Differentially enriched virulence factors were identified by using Kruskal–Wallis test. Microbial community types (enterotypes) The community type of each faecal metagenomic sample was analyzed by the PAM-based method using relative abundances of genera [16] , [19] , and by the Dirichlet multinomial mixture model-based method using counts of sequencing reads [20] ( Supplementary Methods ). Metagenome-wide association study (MGWAS) For comparison of the faecal microbiome in healthy controls, advanced adenoma and carcinoma patients, genes that showed significant difference in relative abundance between any of the two groups were identified (Benjamin–Hochberg q -value<0.1, Kruskal–Wallis test). These marker genes were then clustered into MLGs according to their abundance variation across all three groups of samples [16] . Nine of the 147 samples contained >20% Escherichia (2 controls, 2 adenoma and 5 carcinoma samples), and were only used subsequently in the test sets for the MLG-based adenoma or carcinoma classifiers ( Fig. 5 ). Nine additional samples taken for another manuscript (six healthy controls and three advanced adenoma samples, Supplementary Data 1 ) were also used in the test sets for the classifiers. Taxonomic assignment and abundance profiling of the MLGs were performed according to the taxonomy and the relative abundance of their constituent genes, as previously described [16] . Briefly, assignment to species requires >90% of genes in an MLG to align with the species’ genome with >95% identity and 70% overlap of query. Assigning an MLG to a genus requires >80% of its genes to align with a genome with 85% identity in both DNA and protein sequences. When comparing two groups, for example, controls and adenoma, MLGs were further clustered according to Spearman’s correlation between their abundances in all control and adenoma samples, and the co-occurrence network was visualized by Cytoscape 3.0.2. The direction of enrichment was determined by Wilcoxon rank-sum test ( P <0.05). MLG-based classifier A 10-fold cross-validation was performed on a random forest model (R 3.0.2, randomForest4.6-7 package) using the MLG abundance profile of the control, advanced adenoma or carcinoma samples ( Supplementary Methods ). The cross-validational error curves (average of 10 test sets each) from 5 trials of the 10-fold cross-validation were averaged, and the minimum error in the averaged curve plus the s.d. at that point was used as the cutoff. All sets (≤ 50) of MLG markers with an error less than the cutoff were listed, and the set with the smallest number of MLGs was chosen as the optimal set. The probability of adenoma or carcinoma was calculated using this set of MLGs and an ROC was drawn (R 3.0.2, pROC3 package). The model was further tested on the testing set and the prediction error was determined. PERMANOVA on the influence of clinical and lifestyle factors Permutational multivariate analysis of variance (PERMANOVA) [57] was performed on the gene abundance profile of all samples to assess impact from each of the factors listed ( Supplementary Methods ). We used Euclidean distance and 9,999 permutations in R (3.0.2, vegan package [58] ). Canonical correspondence analysis Canonical correspondence analysis was performed on the MLG (>100 genes) abundance profile of the control, adenoma and carcinoma samples together to assess impact from each of the factors listed ( Supplementary Methods ). The plot was generated by R (3.0.2, vegan package [58] ). KEGG analysis Putative amino acid sequences were translated from the gene catalogues and aligned against the proteins/domains in the KEGG databases (release 59.0, with animal and plant genes removed) using BLASTP (v2.2.24, default parameter except that -e 0.01 -b 100 -K 1 -F T -m 8). Each protein was assigned to the KO group by the highest scoring annotated hit(s) containing at least one HSP scoring >60 bits. Differentially enriched KO modules were identified according to their reporter score [59] from the Z -scores of individual KOs. One-tail Wilcoxon rank-sum test was performed on all the KOs that occurred in more than five samples and adjusted for multiple testing using the Benjamin-Hochberg procedure. The Z -score for each KO could then be calculated: where θ −1 is the inverse normal cumulative distribution, is the adjusted P value for that KO. The aggregated Z -score for a KEGG pathway (or module) is then: where k is the number of KOs involved in the pathway (or module). We corrected the background distribution of Z pathway by subtracting the mean ( μ k ) and dividing by the s.d. ( σ k ) of the aggregated Z -scores of 1,000 sets of k KO, chosen randomly from the whole metabolic KO network: The Z adjustedpathway was used as the final reporter score for evaluating the enrichment of specific pathways or modules. A reporter score of ≥1.6 (90% confidence according to normal distribution) could be used as a detection threshold for significantly differentiating pathways. Accession codes: The metagenomic shotgun sequencing data for all 156 samples have been deposited to the EBI database under the accession code ERP008729. How to cite this article: Feng, Q. et al . Gut microbiome development along the colorectal adenoma–carcinoma sequence. Nat. Commun. 6:6528 doi: 10.1038/ncomms7528 (2015).